Vibrational dynamics and surface structure of amorphous selenium In contrast to crystalline solids in which structural order governs dynamics and thermodynamics, the lack of long-range periodicity in amorphous materials is responsible for several anomalies. Although the relation between these anomalies and the 'bulk structure' is generally understood, the surface structure and the corresponding vibrational spectrum of amorphous solids is practically an unexplored theme. In this study, we resolve the differences in vibrational dynamics and atomic structure between bulk and surface (top 5 nm) atoms of amorphous selenium. We combine experimental (grazing incidence inelastic X-ray scattering) and computational ( ab initio and semiempirical molecular orbital theoretical calculations) methods to scrutinize a variety of possible structural models. We find that a high concentration of particular types of 'coordination defects' in the surface layer is responsible for the observed differences. Resolving the structure of amorphous surfaces is, for example, important for understanding nanoparticles' properties where the surface–to–bulk ratio has a crucial role. Whereas structural and vibrational properties of crystalline materials can be measured in great detail by various techniques, properties of amorphous materials are much harder to resolve. For this and other reasons, thermal and vibrational properties in amorphous materials have long been a source of controversy [1] , [2] , [3] . However, recently, some progress has been achieved for the 'bulk structure' [4] , [5] , [6] . Vibrational excitations at ordered surfaces have methodically been studied for several decades, both experimentally and theoretically [7] . These studies have mainly provided an insight into the nature of the bonding between atoms of a crystalline solid and adsorbates, that is, molecules chemisorbed at surfaces and the underlying solid. Until now, the main experimental tools of surface vibrational excitations have been electron energy loss spectroscopy [7] and inelastic helium atom scattering [8] . Despite some recent pioneering experiments on the surface vibrational properties of amorphous silica [9] , [10] , almost nothing is known about the surface structure and the corresponding surface vibrational properties of an amorphous solid itself. On the other hand, recent studies of surface relaxation dynamics in glasses revealed significant differences between bulk and surface relaxation [11] , [12] at temperatures below the glass transition temperature, T g . The existence of a liquid-like layer, several nanometres thick, at the surface of a polymer glass at T < T g , differentiating surface from bulk dynamics has been suggested [12] . Because of the absence of nearest neighbours on the vacuum side, atoms at or near the surface experience an anisotropic field of interatomic forces. As a result, atoms near the surface of crystalline materials assume positions with different spacing and/or symmetry from the bulk atoms. The change in equilibrium positions near the surface can either be a purely normal relaxation (where the surface layer contracts as a whole towards the bulk) and/or a reconstruction (where the two-dimensional (2D) structure of the surface alters). Whereas in the latter case, atoms in the surface layer rearrange their bonds (often trying to attain the same coordination number as in the bulk), no bond rearrangement takes place in the case of a pure relaxation. As a consequence, the top-most surface atoms are less coordinated than bulk atoms. Note that, in contrast to the conventions used in solid-state physics, this is not called a 'coordination defect' in surface science. In practice, only deviations from the normal surface-bonding situation (as for example at steps, kinks and so on) are named 'coordination defects' in surface science. Contrary to crystalline solids, amorphous materials do not reconstruct in a regular and well-ordered manner, but surface deviations are substantiated by randomly distributed coordination defects, that is, changes in the coordination number of a given atom. Resolving structure and vibrational properties at surfaces will have implications in understanding not only their physical properties but also similar properties of nanoparticles where the surface-to-volume fraction of atoms is significant. In particular, the functionality of the surfaces (1–3 nm thick) has implications for semiconductor device fabrication, catalysis, self-assembled monolayers and so on [7] . It is now well established that, when considered from the viewpoint of vibrational dynamics, crystalline and non-crystalline materials exhibit noticeable differences in their vibrational density of states (VDoS), g ( E ) [13] . The lack of long-range periodicity is responsible for the universal presence, in non-crystalline solids, of low-energy excitations in excess to the counterpart crystal [13] . The specific energy range where such excitations arise is weakly material dependent, always lying in the range 0.3–1 THz. Low-energy excitations account for several properties, including the specific heat excess (bump in the C ( T )/ T 3 plot) at temperatures around 5–10 K, the plateau in thermal conductivity at about the same temperature, and the presence of scattering intensity in Raman and inelastic incoherent neutron-scattering spectra (Boson peak), in excess to the Debye prediction g D ( E ) [13] , [14] , evidenced as a peak in the reduced g ( E )/ E 2 . Actually, recent detailed analysis of several experimental data revealed that the true excess VDoS, g D ( E )− g ( E ), conveys much more useful information, than the reduced form, about the changes of excess modes under the application of external stimuli, such as temperature, pressure, light illumination and so on [15] . Inelastic X-ray scattering (IXS) over the last decade has proven to be a very valuable tool in studying amorphous materials. Despite the lack of periodicity in such materials, the presence of phonon-like excitations in glasses has been documented in IXS experiments [16] . These are manifested by the presence of dispersion relations that persist up to wavevectors' magnitudes, Q , which are a significant fraction of the first maximum of the static structure factor, S ( Q ) [16] . An additional advantage of IXS is that in the high- Q limit, where the static structure factor approaches a constant value, it allows determining the VDoS of a disordered material [17] (incoherent approximation). In addition, as total external reflection of X-rays occurs below a certain angle, the VDoS of a glass surface can be measured under grazing incidence conditions. Inelastic (Raman) scattering can also delineate the qualitative features of VDoS; however, the involvement of the frequency-dependent light-to-vibration coupling function makes the quantitative determination of the relative band intensities not straightforward. Alternatively, the VDoS of limited size clusters of atoms can be determined by ab initio quantum chemical calculations. However, because this method is effective only for small clusters of atoms due to computer program limitations in the calculation of the VDoS, ab initio molecular dynamics simulations are usually employed instead [4] . Semiempirical quantum mechanical calculations are also robust and accurate in the determination of structure and vibrational spectrum, furthermore having the advantage of providing the VDoS of clusters much larger in size than those calculated by ab initio methods. Here, we present the experimental determination of the VDoS of amorphous selenium (a-Se) using IXS in both the bulk and the surface-sensitive geometries. The IXS experiment was performed at the ID28 beam-line of the European Synchrotron Radiation Facility (ESRF), exploiting the nine analysers for simultaneous multi- Q data acquisition. To understand the structural origin of the observed difference between the bulk and the surface VDoS, we carried out ab initio and semiempirical quantum mechanical calculations for structural models of a-Se of various sizes. Thus, here, we identify the nature of the coordination defects in the surface layer, which are responsible for the appearance of gap modes in the surface v-DoS as compared with the bulk v-DoS. 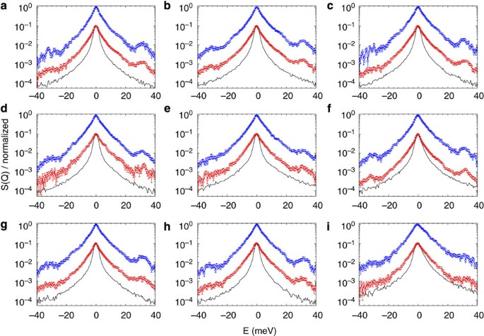Figure 1: Bulk and surface structure factors of a-Se. Fixed momentum transfer spectra for the nine analysers presented in a semilogarithmic scale. The wavevectors of the nine analysers correspond to following values: (a) 44.36 nm−1, (b) 46.68 nm−1, (c) 48.99 nm−1, (d) 51.30 nm−1, (e) 53.59 nm−1, (f) 45.49 nm−1, (g) 47.81 nm−1, (h) 50.11 nm−1, (i) 52.40 nm−1. The bulk glass data are indicated by blue squares and the surface-sensitive geometry data by red circles (data divided by a factor of 10). The solid black line represents the instrument resolution for each analyser. The observed features are discussed in the text. Error bars, which represent the s.d. of the data, are shown for the bulk and the surface data points. Experimental VDoS for bulk and surface-sensitive geometries Representative structure factors S ( Q , E ) collected at fixed momentum transfer are presented in Figure 1 . Comparing the spectral profile of the instrumental resolution function (solid curve) with the measured spectra for all wavevectors, it is seen that the S ( Q , E ) exhibit predominant contributions from elastically scattered photons. However, inelastic features superimposed onto the elastic peak are clearly discernible at ∼ 15 and ∼ 32 meV. From the measured S ( Q , E ) spectra, the VDoS can be extracted using the analysis described in the Methods section. In brief, the Wiener deconvolution algorithm [18] was used to remove the effect of the instrumental function. 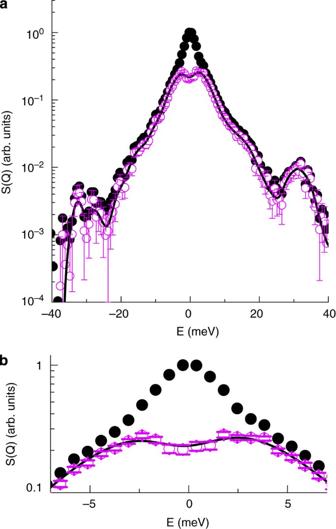Figure 2: Wiener-filter analysis of measured structure factors. (a) Performance demonstration of the Wiener-filter algorithm as used in the data analysis. The recordedS(Q,E) spectra are broadened owing to the finite width of the instrument functionfinstr. As the instrument function is known,S(Q,E) can be recovered by the Wiener deconvolution algorithm. The unconvoluted spectra forS(Q,E•Figure 2 | (a) Performance demonstration of the Wiener-filter algorithm as used in the data analysis. The recorded S(Q, E) spectra are broadened owing to the finite width of the instrument function finstr. As the instrument function is known, S(Q, E) can be recovered by the Wiener deconvolution algorithm. The unconvoluted spectra for S(Q, E) (filled circles) analyser 1 of the bulk data) andS(Q,E) after subtraction of the elastic line (open circles) are plotted. The solid line representsS(Q,E) after the application of the Wiener filter re-convoluted with the instrument function. (b) Close-up of the low-energy region of panela. In both panels, the error bars plotted forS(Q,E) after subtraction of the elastic line (open circles) represent the s.d. of the data. The reliability of the algorithm's application to the present data is demonstrated in Figure 2 . The VDoS were determined under the incoherent approximation using the structural factors at all available values of Q , assuming that single-phonon scattering is predominant. 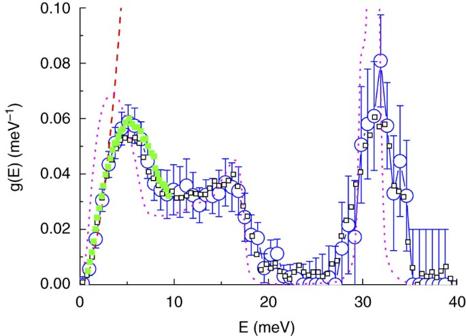Figure 3: Bulk VDoS. Obtained bulk IXS VDoS (open circles) compared with inelastic neutron-scattering data (filled squares: measured at 300 K19, open squares: measured at 100 K20) and molecular dynamics simulations21(dotted line). The Debye limit is indicated by the dashed line. The error bars represent the s.d. of the data. The comparison between the VDoS determined by IXS and inelastic neutron-scattering experiments [19] , [20] and molecular dynamics simulations [21] is shown in Figure 3 for bulk glassy Se. A good agreement has been achieved by selecting an elastic peak contribution of ∼ 60%. Figure 1: Bulk and surface structure factors of a-Se. Fixed momentum transfer spectra for the nine analysers presented in a semilogarithmic scale. The wavevectors of the nine analysers correspond to following values: ( a ) 44.36 nm −1 , ( b ) 46.68 nm −1 , ( c ) 48.99 nm −1 , ( d ) 51.30 nm −1 , ( e ) 53.59 nm −1 , ( f ) 45.49 nm −1 , ( g ) 47.81 nm −1 , ( h ) 50.11 nm −1 , ( i ) 52.40 nm −1 . The bulk glass data are indicated by blue squares and the surface-sensitive geometry data by red circles (data divided by a factor of 10). The solid black line represents the instrument resolution for each analyser. The observed features are discussed in the text. Error bars, which represent the s.d. of the data, are shown for the bulk and the surface data points. Full size image Figure 2: Wiener-filter analysis of measured structure factors. ( a ) Performance demonstration of the Wiener-filter algorithm as used in the data analysis. The recorded S ( Q , E ) spectra are broadened owing to the finite width of the instrument function f instr . As the instrument function is known, S ( Q , E ) can be recovered by the Wiener deconvolution algorithm. The unconvoluted spectra for S ( Q , E •Figure 2 | (a) Performance demonstration of the Wiener-filter algorithm as used in the data analysis. The recorded S(Q, E) spectra are broadened owing to the finite width of the instrument function finstr. As the instrument function is known, S(Q, E) can be recovered by the Wiener deconvolution algorithm. The unconvoluted spectra for S(Q, E) (filled circles) analyser 1 of the bulk data) and S ( Q , E ) after subtraction of the elastic line (open circles) are plotted. The solid line represents S ( Q , E ) after the application of the Wiener filter re-convoluted with the instrument function. ( b ) Close-up of the low-energy region of panel a . In both panels, the error bars plotted for S ( Q , E ) after subtraction of the elastic line (open circles) represent the s.d. of the data. Full size image Figure 3: Bulk VDoS. Obtained bulk IXS VDoS (open circles) compared with inelastic neutron-scattering data (filled squares: measured at 300 K [19] , open squares: measured at 100 K [20] ) and molecular dynamics simulations [21] (dotted line). The Debye limit is indicated by the dashed line. The error bars represent the s.d. of the data. Full size image The same analysis was then applied to the data recorded in surface-sensitive geometry. 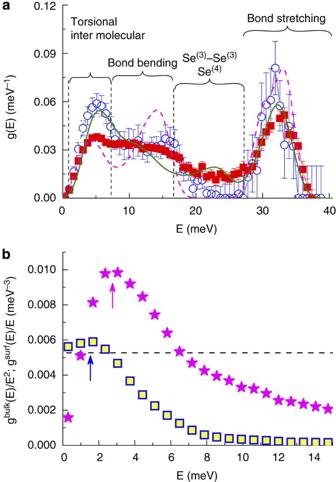Figure 4: Experimental and simulated VdoS. (a) VDoS of a-Se measured in bulk (open circles) and surface-sensitive geometries (filled squares). The gap that separates acoustic and optic modes in the bulk disappears at the surface. The solid and dashed lines represent, respectively, the simulated VDoS of the surface () and bulk () structural models. The areas of all curves are normalized to unity. Error bars, indicated for the measured bulk and surface VDoS, represent the s.d. of the data. (b) Reduced VDoS (Boson peaks) for the bulk (squares, divided byE2) and surface (stars, divided byE) experimental data. The Debye limit of the bulk glass is shown by the dashed line. In Figure 4a, the VDoS obtained in surface-sensitive, g surf ( E ), and bulk-sensitive, g bulk ( E ), geometries are presented and compared. Two main differences can be made out from this comparison. At low energy (between 2 and 8 meV), a reduction in the density of vibrational modes is observed in the surface VDoS in comparison with the bulk one. In the region from 17 to 28 meV, the gap that separates acoustic and optic modes in the bulk VDoS is filled with new vibrational states in the surface VDoS. A further difference between bulk and surface v-DoS is emphasized by comparing the Boson peak (determined as g bulk ( E )/ E 2 and g surf ( E )/ E , respectively), which is located at 1.7 meV in the bulk and shifts to ∼ 2.8 meV in the surface ( Fig. 4b ). Figure 4: Experimental and simulated VdoS. ( a ) VDoS of a-Se measured in bulk (open circles) and surface-sensitive geometries (filled squares). The gap that separates acoustic and optic modes in the bulk disappears at the surface. The solid and dashed lines represent, respectively, the simulated VDoS of the surface ( ) and bulk ( ) structural models. The areas of all curves are normalized to unity. Error bars, indicated for the measured bulk and surface VDoS, represent the s.d. of the data. ( b ) Reduced VDoS (Boson peaks) for the bulk (squares, divided by E 2 ) and surface (stars, divided by E ) experimental data. The Debye limit of the bulk glass is shown by the dashed line. Full size image Computational-aided evaluation of defects in a-Se To understand the nature of the experimentally observed differences between the bulk and the surface VDoS, ab initio and semiempirical calculations based on molecular orbital theory were employed for various Se clusters containing coordination defects. At the outset, Se 6 and Se 8 rings, vibrational features of which are accurately known from Raman scattering experiments [22] , [23] , were calculated by both methods ( Supplementary Fig. S1 ). In view of the very good agreement between these two approaches (see the geometrical details and vibrational frequencies in Supplementary Table S1 ), the semiempirical method was subsequently used to study the structure and vibrational modes of much larger structural models of a-Se, providing information beyond the capabilities of ab initio calculations. Comparison between experiments and calculations ( ab initio and semiempirical methods) provides a common scaling factor (0.86) that has to be applied in order to bring the calculated and experimental frequencies in coincidence ( Supplementary Fig. S2 ). Evidently, defective atomic-bonding arrangements of a-Se must be invoked to account for the appearance of extra vibrational modes in the gap of the VDoS ( Fig. 4a ). The existence of defects at surfaces is a well-known fact. A frequent type of defect is related to deviations from the coordination number dictated by the valence electrons [1] . Normal bonding in a-Se requires that Se atoms are two-fold coordinated forming mostly ( ∼ 90% of atoms) long helical chains and partly ( ∼ 10% of atoms) Se 8 rings, as revealed by recent high-resolution, off-resonant Raman scattering [24] . Three-fold-coordinated Se atoms, Se (3) , have been frequently invoked as structural 'defects' arising either from illumination with proper light energy in a-Se films [25] or naturally from the bulk liquid phase [26] . The appearance of a new bond at a Se atom that has already satisfied its bonding requirements (8- N rule) implies a redistribution of the electronic density, hence causing weakening of the covalent bonds. Efforts are, therefore, focused on the types of the possible defects that can appear in a-Se. The one-dimensional (1D) nature of Se chains (dictated by the low coordination number of Se) limits the types of defects to the following candidates: one-fold (undercoordinated) terminal Se atoms, three-fold (overcoordinated) Se atoms, valence alternation pairs of one-fold and three-fold-coordinated Se atoms, pairs or clusters of three-fold-coordinated atoms, and four-fold (overcoordinated) Se atoms. A detailed analysis of Se clusters of various sizes and geometries revealed that only pairs or clusters of three-fold Se atoms' and four-fold Se atoms' hypervalent defects possess vibrational modes situated in the energy gap ( Supplementary Figs S3–S8 ). Interestingly, calculations showed that the bond lengths of single or isolated Se (3) atoms (three-fold Se surrounded only by two-fold Se atoms) were not appreciably different than the bond lengths of the normal two-fold or Se (2) atoms ( Supplementary Fig. S3 ). As a result, the calculated vibrational frequencies of the Se (3) –Se (2) bond were found in the spectral range of the bond-stretching band ( E >28 meV). However, when two Se (3) atoms share a common bond, forming Se (3) –Se (3) pairs, ( Supplementary Fig. S4 ) calculations revealed that this bond is indeed longer (weaker) than bonds between two-fold Se atoms. Therefore, the vibrational frequency of this long bond falls within the gap of the bulk VDoS ( Supplementary Fig. S5 ). The aforementioned hypervalent defects are evident in the simulation of a large cluster of 96 Se atoms. 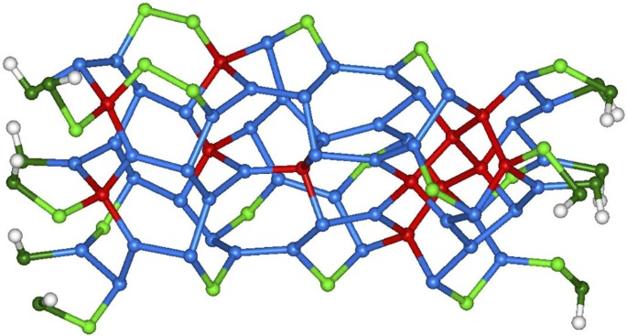Figure 5: A 96-atom a-Se structural model. Ball and stick representation of a fully optimized 96-atom Se structural model representing the outermost skin of a-Se surface. Coloured atoms description is as follows: light green, two-fold Se; dark green, Se atom terminated by H-bond; blue, three-fold Se; red, four-fold Se; grey, H atom. The starting configuration is shown in Supplementary Figure S7a and the optimized geometry is illustrated in Figure 5 . The calculated vibrational spectrum of this 96-atom Se structural model, , is shown in Figure 4a (solid line). For comparison, the corresponding spectrum of a 96-atom Se helical chain, , which is a reasonably good representation of bulk Se structure, is also shown (dashed line). The spectra are constructed using Gaussian distribution broadening (3 meV full-width) to account for the inhomogeneous broadening in the amorphous state and hence to facilitate the comparison with the experimental spectra. Figure 5: A 96-atom a-Se structural model. Ball and stick representation of a fully optimized 96-atom Se structural model representing the outermost skin of a-Se surface. Coloured atoms description is as follows: light green, two-fold Se; dark green, Se atom terminated by H-bond; blue, three-fold Se; red, four-fold Se; grey, H atom. Full size image The calculated VDoS of the cluster, shown in Figure 4a , bears a remarkable resemblance with the experimental surface VDoS. It shows, in particular, the new modes appearing in the gap, the spectral form of which is qualitatively, and partly quantitatively, similar to the experimental one. The theoretical VDoS exhibits a local maximum at ∼ 21 meV. Analysis of the calculated frequencies revealed that this bump in the VDoS is related to a medium range structural motif, where a hypervalent atom is surrounded exclusively by other hypervalent atoms. An important finding of the simulation is that—in accordance with the experimental data—the part of the bulk VDoS that accounts for bond-bending vibrations is depleted in the VDoS of . In this context, it is interesting to note that first-principles molecular dynamics simulations [26] suggested that pairs of three-fold Se (3) and Se (4) atoms are the dominant defects in liquid Se. It was also found that Se (3) atoms exhibit a high tendency to cluster together in liquid Se. Almost 82% of three-fold Se atoms were found to occur in the form of Se (3) –Se (3) pairs [26] , that is, in the special defect configuration, which our analysis showed that its vibrational frequency falls within the gap of the VDoS. Apart from accounting for the new modes in the VDoS gap, hypervalent defects, Se (3) –Se (3) pairs and Se (4) , can also provide a rationale for the depletion of the torsional and interchain part observed in the surface VDoS. Se chain interconnection implies change of the local dimensionality from 1D to quasi-2D or even three-dimensional (3D; locally), see Figure 5 . Apparently, the low-energy floppy modes (intrachain torsional motions and interchain vibrations of chains interacting weakly by means of van der Waals forces) are prohibited when chains become interconnected, rendering the system more rigid. Torsional motions involve rotational-like motion or changes in the dihedral angle defined by four-atom arrangements. The overconstrained parts of chains (due to hypervalent defects) do not allow such motions to occur and hence the relevant part of the surface VDoS in the energy range 3–8 meV appears weaker in comparison with the bulk one. The different topological order and the increased stiffness of the surface (owing to a high density of overcoordinated Se atoms) in comparison with the bulk properties are also reflected in the Boson peak spectral features. As Figure 4b shows, the Boson peaks for the bulk glass and the amorphous surface, determined as g bulk ( E )/ E 2 and g surf ( E )/ E , respectively, exhibit appreciable differences. Most notably, the surface Boson peak appears at ∼ 2.8 meV being appreciably different compared with the bulk Boson peak situated at 1.7 meV. This observation is in accord with the generally accepted context that the Boson peak energy increases when the glass becomes stiffer (increase of elastic constants). However, at this point, a discussion of the enhanced intensity of the surface Boson peak would be highly speculative; however, the amount of excess surface states critically depends on the knowledge of the surface Debye level, a quantity which has not yet been determined for a-Se. To our knowledge, a-Si is the only non-crystalline solid the surface structure of which has been systematically examined by computer simulations. In line with our findings, simulation studies of a-Si surfaces have revealed coordination defects deviating from the normal four-fold coordination of Si atoms. Two main types of defects are frequently found: three-fold (undercoordinated) Si atoms with dangling bonds and five-fold (overcoordinated) Si atoms with floating bonds. The first theoretical study of the surface structure of a-Si concluded that both dangling bonds and floating bonds exist on the surface with the former being more probable [27] . In a more recent thorough simulation study, it was found that the details of the interatomic potentials determine the ratio of three-fold and five-fold-coordinated Si atoms [28] . The difference in the electronic structure between Si and Se is responsible for the higher 'structural contrast' between bulk and surface structures in a-Se in comparison with a-Si. The 3D structure of bulk a-Si is practically not altered on the surface by removing or adding one bond. On the contrary, the 1D nature of the a-Se chains is severely altered either to 2D due to three-fold Se bonding or even to 3D (locally) due to four-fold hypervalent defects, adding an extra rigidity on the surface layer. The change (increase) in the coordination number of Se atoms on the surface in comparison with the bulk value discloses one way of how strain can be accommodated by amorphous surfaces. While surface relaxation and reconstruction of crystalline solids affects only the top-most layers of atoms, strain release in a-Se involves a surface thickness of a few nanometres. We anticipate that this might be a result of broader validity: the amorphous structure seems to convey surface strain much more easily into the bulk than crystalline materials. Apart from other glasses, this has also implications for the understanding of nanoparticles where the surface-to-bulk ratio is important. Studies of the vibrational dynamics of glassy nanoparticles could shed light on the nature of the Boson peak as well as on low-temperature anomalies of thermal properties (for example, heat capacity and thermal conductivity). In conclusion, the present joint experimental and theoretical study revealed that hypervalent defects (pairs of three-fold and four-fold Se atoms) form medium-range structural order motifs that are responsible for the appearance of modes in the gap of the VDoS. This branching of the 1D Se chains leads to the formation of a 'protective' surface layer of the material, few nanometres in thickness with enhanced rigidity, which can affect the functionality and responsiveness of the surface. The enhanced rigidity of the protective surface layer in a-Se has to be contrasted to the liquid-like layer that exists on crystalline ice surfaces where a liquid-like layer appears even at temperatures below the melting point [29] . Although thermodynamic and elastic properties of macroscopic objects are largely determined by the bulk VDoS, the surface contribution to the VDoS becomes significant for materials with a high surface-to-bulk fraction, for example, silica gel, foams and nanoparticles. In this context, it would be appealing to study how the VDoS is affected by systematically increasing the surface-to-bulk ratio. Sample preparation Two different methods were used to prepare non-crystalline Se samples. Amorphous Se thin films ( ∼ 1 μm in thickness) on Si substrates were prepared for the surface-sensitive experiments by pulsed laser deposition. A KrF laser (Lambda Physik COMPex 102) operated at 248 nm with constant output energy of 200 mJ per pulse (pulse duration of 30 ns, repetition rate of 20 Hz, energy density was 1 J cm −2 and beam spot dimension was 1×1 mm 2 ) was employed. The laser beam was focused by a spherical lens (focal length 0.61 m) on the target (bulk glassy Se) at an incidence angle of 45° normal to the target surface. The target-to-substrate distance was 50 mm. The pulsed laser deposition experiments were performed at 4.7×10 −4 Pa pressure for time duration of 24 min. Particular care was taken to keep the sample surface clean at all stages. The a-Se films were sealed under vacuum in Pyrex tubes for the shipment to ESRF and for storage before the experiment. On site, the sample was transferred into an ultra-high vacuum (UHV) pocket cell. The procedure took place in an Ar-filled glove box. Thereafter, the Ar inside the pocket cell was replaced by He and a constant He flow was adopted throughout the experiment. For the experiments where the bulk VDoS is measured, a thick ( ∼ 40 μm) glassy Se flake was produced by melt quenching (hot pressing of liquid Se on stainless steel surface in inert atmosphere). The Se flake was attached to a copper holder with a proper pinhole. The sample thickness was chosen to match the absorption length at the incident energy of 17,794 eV, which corresponds to the (9 9 9) reflection from the silicon analyser that we utilized ( δE ≈3 meV). IXS experimental details and data analysis IXS spectra were recorded at selected scattering angles, which correspond to fixed momentum transfers covering the Q -range 44.36< Q <52.40 nm −1 . A typical acquisition time for one energy scan (−40< E <40 meV, 150 s per data point) was about 5 h, and the scans were repeated for a total integration time of about 300 s per point. The surface sensitive geometry is achieved by working at grazing incidence conditions below the critical angle of total reflection, α c . In this configuration, the electromagnetic radiation is totally reflected, however, an evanescent wave travels along the surface boundary. For the chosen incident angle of 0.6× α c =0.079°, the topmost 5 nm of the a-Se film is probed. Proper alignment of the incident X-ray beam was checked by verifying that no phonons of the Si substrate appeared in the measured spectra. If the beam is not perfectly aligned (for example, because of an incident angle > α c ), then the X-rays also penetrate into the Si substrate. In this case, apart from the S ( Q ) of the Se film, one observes distinct acoustic phonons of the Si substrate. As in the present experiment nine analysers are simultaneously employed at different Q values, these phonons can easily be distinguished from the VDoS of the Se-film owing to their Q -dispersion. The manipulation of the raw data took place as follows. First, we performed background subtraction from each spectrum and normalization to S ( Q ) to get rid of all the Q- dependent factors, such as detector efficiencies, polarization dependence and form factor. This yields the dynamic scattering factor S ( Q , E ), which contains contributions from elastic scattering as well as from single-phonon and multiphonon interactions of the scattered photons, convoluted with the resolution function of the instrument f inst . Here S n ( Q , E ) represents the scattering factors for n =0, 1, 2, ... phonon interactions and the symbol ⊗ denotes the convolution with the instrument function. The deconvolution of S *( Q , E ) ⊗ f inst is achieved using the Wiener deconvolution algorithm [18] , that is, an application of the Wiener filter to the noise problems inherent in deconvolution. The asterisk in the structure facture indicates the purely inelastic scattering contributions, that is, the absence of the n =0 phonon interactions in equation (1). The algorithm works in the frequency domain, attempting to minimize the impact of convolution created by noise at frequencies that have a low signal-to-noise ratio. The S *( Q , E ) function obtained after applying the Wiener deconvolution was checked by convolution with the instrument function; the resulting signal is practically identical to the original spectrum, see Figure 2 . Having determined S *( Q , E ), a first estimate of the VDoS can be obtained by summing up the signals of all the available analysers corresponding to different Q , that is, using the so-called incoherent approximation, and assuming that single-phonon scattering is predominant S *( Q , E )≈ S 1 ( Q , E ). Within these approximations, the VDoS can be determined by: where the term is the Bose–Einstein distribution for annihilation and creation events. On the basis of this first estimate of the VDoS, the multiphonon analysis by Sjolander [30] can be performed to get the genuine one-phonon contribution S 1 ( Q , E ) out of S *( Q , E ) by an iterative procedure. The dynamic structure factor can be written as: where 2 W is the Debye–Waller factor. The value of 2 W is obtained from the ratio of the elastic to total scattered intensity. The functions G n ( E ) are normalized to unity and are given by with where γ (0)=6 T /Θ Debye , where Θ Debye is the Debye temperature. The constant A that appears in equations (3) and (4) contains physical constants, the scattering cross section, the effective scattering mass and the Debye temperature. It is most easily determined by the ratio of S 1 ( Q , E ) to (2 W × G 1 ) by virtue of equation (3). For increasing n , a better estimate of the single-phonon scattering factor S 1 ( Q , E ) can now be obtained iteratively by making use of equations (2), (4),(5),(6),(7),(8). Inserting the VDoS obtained from equation (2) into equation (8) yields from which the two-phonon contribution G 2 ( E ) is obtained according to equation (6). Subsequent subtraction of the two-phonon contribution from S *( Q , E ) in equation (4) leads to an improved S 1 ( Q , E ). With this new S 1 ( Q , E ), the above steps are repeated for increasing n , thus taking interactions of more and more phonons into account. The iteration terminates when numerical convergence of S 1 ( Q , E ) is achieved. Best agreement of the bulk VDoS measured by IXS and inelastic neutron-scattering experiments [19] , [20] is achieved for an elastic peak contribution of a 0 =0.6, see Figure 3 . Simulation method Simulations of Se 6 and Se 8 rings with accurately known vibrational frequencies from experiments revealed that both ab initio and semiempirical methods provide a common scaling factor (0.86), which has been applied in the present article, to bring calculated and experimental frequencies in coincidence ( Supplementary Fig. S2 ). This finding demonstrates that semiempirical calculations (at the level of the theory we employed) are capable of providing an accurate determination of the vibrational frequencies of larger structural models of elemental Se. On the basis of this finding, a 96-atom Se single chain ( ) and six 16-atom Se chains in parallel arrangement ( ), see Supplementary Figure S7a , were used as the starting configurations to simulate the structure of the bulk and the outermost surface skin layer of a-Se, respectively. H atoms have been added to the Se chains ends to account for finite size effects. The Hartree–Fock molecular orbital theoretical approach, as implemented in the GAUSSIAN03 programme package [31] , was employed for calculating the vibrational properties of the ring structures (Se 6 and Se 8 ). The basis set that has been used is the valence triple zeta + polarization [32] . The initial basis set (14s11p5d) is contracted to (8s6p2d). A polarization d-function was added leading to the final basis set (8s6p3d) [33] . The semiempirical level of molecular orbital theory, developed under the Hartree–Fock theory using various approximations, was used to simulate and . The method provides a useful tool to understand and/or predict the structure and the properties of various chemical systems, which consist of a large number of atoms. Semiempirical methods have been extensively used in the past years to treat large systems and complicated processes, because of their computational efficiency [34] . Although their setup is derived from Hartree–Fock theory, the design of approximate energy expressions and the empirical parameters are used to achieve higher accuracy than the underlying ab initio theory [34] . The accuracy of semiempirical methods is based on the comparison of the calculated values of the molecular properties with the experimental and high-level ab initio or density functional theory values. Specifically, in the computational part of our study, the calculations were performed with the parametric method 6 [35] included in the version 2009 of MOPAC programme package (MOPAC2009, Stewart Computational Chemistry, version 9.055W). This method is based on the neglect of diatomic differential overlap formalism and has very low average errors [32] . The geometries were fully optimized in Cartesian coordinates (XYZ) using the Baker's Eigenvector following routine. As in all quantum mechanical simulations, the semiempirical method, although quite accurate for molecular systems, should be considered with care when used to calculate structure and properties of extended systems, especially when non-periodic structures are studied. In the present case, however, our parametric method 6 studies have a rather comparative character. Our efforts are concentrated on the difference between the bulk structure (long helical chain) and structures containing various defects. Therefore, any systematic errors of the simulation are not expected to severely affect the obtained conclusions; see Supplementary Methods for details. How to cite this article: Scopigno, T. et al . Vibrational dynamics and surface structure of amorphous selenium. Nat. Commun. 2:195 doi: 10.1038/ncomms1197 (2011).